Adaptive sex allocation in anticipation of changes in offspring mating opportunities Sex allocation theory explains why most species produce equal numbers of sons and daughters, and highlights situations that select for deviation from this norm. Past research has, however, heavily focused on situations with discrete generations. When temporally varying generational overlap affects future mate availability, models predict cyclical shifts in sex allocation, but these predictions have not yet been appropriately tested. Here we provide evidence that mosquitofish ( Gambusia holbrooki ) populations possess a suitable life history: some autumn-born females bred alongside their own offspring, while such overlap was rare or absent for spring-born females and for all males. Our analytic model of sex allocation for these populations produced a perfect rank-order correlation between observed birth sex ratio biases and theoretical predictions, with stronger biases observed as the extent of female generational overlap increased. This is the first robust evidence that sex allocation theory accounts for cases when mating opportunities vary predictably over time. In the majority of studied taxa, sons and daughters are produced in equal numbers, that is, a birth sex ratio (BSR; proportion sons) of 0.5 (refs 1 , 2 ). Early sex allocation theory was formulated to explain why this occurs: an overproduction of one sex is balanced by a reduction in the average fitness pay-off for individuals of that sex [3] , [4] . Sex allocation theory, however, also highlights situations that select for deviation from this norm [5] , [6] . Given the preponderance of equal investment, empirical tests are thus most powerful in these situations [5] . Encouragingly, many empirical findings closely match precise theoretical predictions [7] , [8] . Past research has, however, heavily focused on situations with discrete generations [5] , despite suggestions that generational overlap can strongly affect optimal sex allocation [6] . Under most circumstances, adult mortality should not affect sex allocation [9] . This is because the total reproductive output of males and females must always be equal [10] . Thus, whenever an individual dies, the average reproductive output of the remaining individuals of that sex increases. In this way, the expected benefit of producing either a son or daughter is unaffected by adult mortality. However, Werren and Charnov [6] first noted that if the pattern of sex-specific mortality differs across cohorts, there will then be predictable variation in mating opportunities. This, in turn, should favour parents who successfully ‘anticipate’ higher or lower future mating opportunities for sons and bias sex allocation accordingly. Thus, in general, when an offspring’s sex and the timing of its birth interact to influence the degree to which generations overlap, sex biases can become adaptive. Werren and Charnov [6] produced a model of seasonal differences in male mating opportunities that predicts cyclical shifts in sex allocation. It has therefore been known for three decades that sex-biased mortality in one generation can theoretically be ‘taken advantage of’ by biasing sex allocation in the opposite direction in the preceding generation. Surprisingly, however, there have been no robust empirical tests of this prediction, nor have the details of the theory ever been fully presented [5] . A relevant test arises when the sexes differ in generational overlap owing to seasonal changes in sex-specific mortality. Here, we provide evidence that mosquitofish ( G. holbrooki ) populations possess a suitable life history: some autumn-born females bred alongside their own offspring, while such overlap was rare or absent for spring-born females and for all males, regardless of season of birth. Furthermore, the extent of this female-only generational overlap differed between populations. We produce an analytic model of sex allocation tailored to the life history of these populations. Finally, we compare the predicted patterns of sex allocation with the BSR of females collected from the wild in spring and autumn. Life-history observations G. holbrooki are small (males: 25 mm, females: 45 mm), live-bearing freshwater fish (family: Poecillidae) native to South-eastern USA, which were introduced to Australia in the 1920s. We studied three feral populations (A, B and C throughout) in Canberra, Australia. Based on fortnightly population sampling (see Methods), we identified strong breeding peaks in spring and autumn ( Fig. 1 ), suggesting that there are two relatively discrete generations each year. We assessed the life history of each population by visual examination of changes in the body length distributions of fish over time ( Fig. 2 ; Supplementary Data ). We could identify distinct cohorts/generations through discontinuities and bimodalities in these distributions. Our data indicate that G. holbrooki differ in male mating opportunities owing to predictable seasonal differences in female reproductive lifespan, as has been previously described in this species [11] , [12] . Over-wintering males participating in spring breeding then appeared to die ( Fig. 2 ). In contrast, some over-wintering females bred twice: in both spring and autumn. Furthermore, the proportion of these females that bred twice (that is, the extent of generational overlap) varied between populations. In population A, few over-wintering females overlapped with the following generation ( Fig. 2a ). Conversely, in population C, many over-wintering females survived such that the breeding population of females in autumn consisted of roughly equal numbers of young and old females ( Fig. 2c ). Population B showed an intermediate level of female-only generational overlap ( Fig. 2b ). 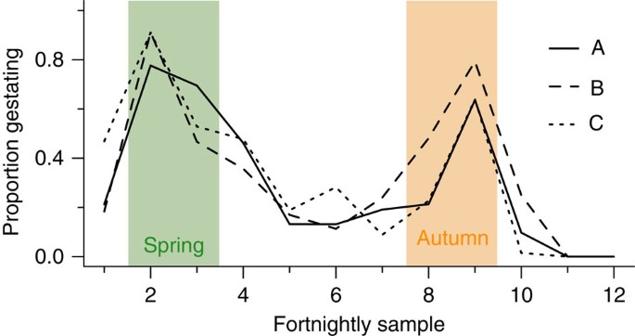Figure 1: Reproductive activity of threeG. holbrookipopulations. Two strong peaks in reproductive activity (indicated by the proportion of females gestating) were seen in all populations in spring (samples 2–3) and autumn (samples 8–9). Figure 1: Reproductive activity of three G. holbrooki populations. Two strong peaks in reproductive activity (indicated by the proportion of females gestating) were seen in all populations in spring (samples 2–3) and autumn (samples 8–9). 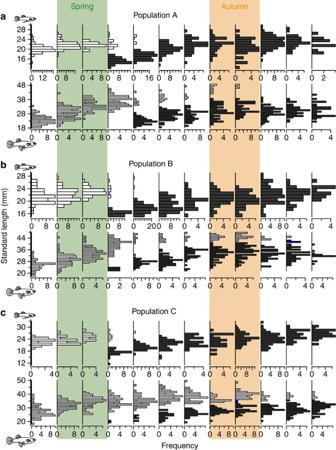Figure 2: Population differences in sex-specific mortality ofG. holbrookias indicated by changes in the length distributions across time. Males (top) and females (bottom) in populations (a) A, (b) B and (c) C. Each histogram is a separate fortnightly sample starting from the left. Spring and autumn-breeding peaks are highlighted. Light bars represent overwintering, autumn-born fish, while dark bars are spring-born fish (based on discontinuity of distributions in standard length and across time). Fish that could not be readily classified are shown in blue. Full size image Figure 2: Population differences in sex-specific mortality of G. holbrooki as indicated by changes in the length distributions across time. Males (top) and females (bottom) in populations ( a ) A, ( b ) B and ( c ) C. Each histogram is a separate fortnightly sample starting from the left. Spring and autumn-breeding peaks are highlighted. Light bars represent overwintering, autumn-born fish, while dark bars are spring-born fish (based on discontinuity of distributions in standard length and across time). Fish that could not be readily classified are shown in blue. Full size image Our data suggest that spring-born fish participate in only autumn breeding and then die; thus only autumn-born fish over-winter (as juveniles). Therefore, we assume that all over-wintering fish were born in autumn. This assumption was made based on the following four lines of evidence. First, in pilot samples in early spring only juveniles were collected in all three populations (although this might be explained by sampling bias if adults are more difficult to catch). Second, the number of adult fish collected in all populations declined markedly from the end of the autumn reproductive peak (sample 9) to the final sample (12) (A: 118–42, B: 126–35 and C: 168–94). Third, there was no evidence of bimodality in the length distributions of over-wintering fish ( Fig. 1 ). Finally, in all cases, over-wintering fish (sample 1) were significantly smaller than fish collected in late autumn (sample 12) that year (Welch’s t -tests, males—A: t 13.8 =2.95, P =0.011, B: t 28.6 =2.28, P =0.030, C: t 57.9 =8.14, P< 0.0001; females—A: t 39.2 =7.64, P <0.0001, B: t 36.9 =4.97, P =0.0002, C: t 120.3 =4.68, P <0.0001). If some or all of the adult breeders in autumn overwintered and continued to grow, we would expect over-wintering fish to be significantly longer than those at the end of autumn (that is, the opposite pattern to that observed), or at least statistically indistinguishable. Thus, multiple lines of evidence suggest that female cohorts of G. holbrooki populations breed once or twice depending on their timing of birth, which implies heightened mating opportunities for spring-born males ( Fig. 3 ). 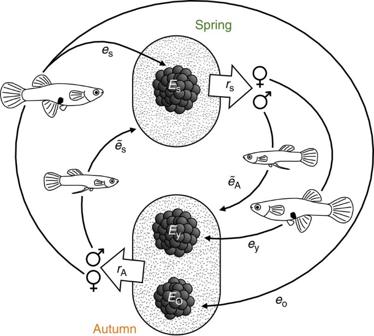Figure 3: Life cycle schematic forG. holbrookipopulations with model parameters. Males born in the preceding season produce sperm (depicted as a ‘cloud’ surrounding eggs) that will fertilize the eggs (E) of these females. The expectedper capitareproductive output of zygotes (e) are depicted graphically by the black arrows. The large white arrows represent sex allocation (r). Populations alternate between one and two cohorts of females breeding simultaneously. Figure 3: Life cycle schematic for G. holbrooki populations with model parameters. Males born in the preceding season produce sperm (depicted as a ‘cloud’ surrounding eggs) that will fertilize the eggs ( E ) of these females. The expected per capita reproductive output of zygotes ( e ) are depicted graphically by the black arrows. The large white arrows represent sex allocation ( r ). Populations alternate between one and two cohorts of females breeding simultaneously. Full size image Analytic model of sex allocation Current tests of sex allocation theory are largely restricted to models assuming a stable age distribution (that is, non-overlapping generations) [5] . Furthermore, the only existing theoretical formulation of anticipatory adjustment of BSRs remains largely verbal [6] . We produced an analytical model of sex allocation for G. holbrooki by considering the total number of eggs ( E ) available to be fertilized at different times and the expected per capita reproductive output of sons ( ë ) and daughters ( e ) in spring and autumn ( Fig. 3 ). Female reproductive success depends on the mean expected number of eggs that each female zygote will go on to produce in spring ( e S ) and autumn ( e Y or e O depending on whether the female is young or old at that time). These values encapsulate both fecundity and survival. For example, if an autumn-born female has poor over-winter survival this lowers her e S as well as e O values, while low survival from spring to autumn lowers her e O only. In spring, the number of eggs available for fertilization ( E S ) is solely attributable to egg production by autumn-born females that have overwintered ( Fig. 3 ). In autumn, the number of available eggs is E Y + E O, that is, those produced by spring-born, young females and by old females that were born the previous autumn, overwintered, bred in spring and then survived to breed again in autumn. Daughters born in autumn have an expected reproductive output of e S in spring and e O in the following autumn. Sons born in autumn only breed in spring with an expected reproductive output of ë S . Daughters and sons that are born in spring only breed in autumn, with expected reproductive outputs of e Y and ë A , respectively ( Fig. 3 ). As we assume that no males survive to breed during both reproductive peaks, male reproductive success equals the mean number of eggs that each male zygote will go on to fertilize during a single reproductive peak ( ë S and ë A in spring and autumn, respectively). This is simply the total number of eggs available ( E ) during each reproductive peak divided by the number of males born during the previous reproductive peak. To then compare the value of producing sons versus daughters for a given reproductive peak, we need to calculate the mean genetic contribution of individuals of each sex to the population at the end of the breeding season. This contribution can arise directly through the production of offspring, or indirectly owing to simultaneous reproduction by a focal individual’s offspring in the same breeding season (that is, production of grandchildren). Using the aforementioned parameters, we derive a series of mathematical relationships for this system (see Methods). We then predict optimal patterns of sex allocation by balancing the expected reproductive values of sons and daughters in each season (details in Methods). The optimal BSR predicted by our analytic model in spring ( r S ) and autumn ( r A ) was: ( E O + E Y )/ ( E O +2 E Y ) and ( E O +2 E Y )/ (4 E O +4 E Y ) respectively ( Fig. 4a ). 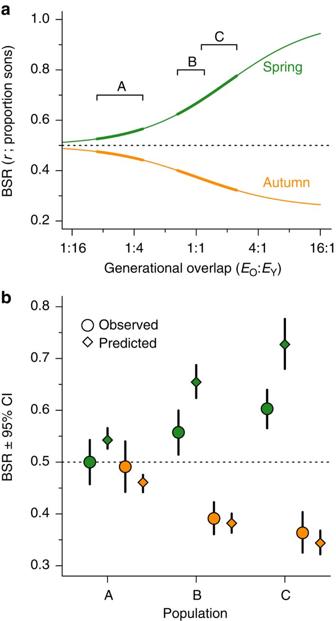Figure 4: Model predictions and observed sex allocation biases. (a) Predicted BSR biases with respect to generational overlap (EO:EY). Separate lines represent optimal sex allocation patterns in spring (rS) and autumn (rA). The bold sections of these lines indicate predictions from our model when it was parameterized with field estimates. (b) Comparison of observed and predicted BSR biases inG. holbrookipopulations. For observed data, the means ±95% confidence intervals are presented. For the predictions, mean and ‘range’ estimates are presented (details in Methods). In both figures, the dotted line represents equal production of sons and daughters. Figure 4: Model predictions and observed sex allocation biases. ( a ) Predicted BSR biases with respect to generational overlap ( E O : E Y ). Separate lines represent optimal sex allocation patterns in spring ( r S ) and autumn ( r A ). The bold sections of these lines indicate predictions from our model when it was parameterized with field estimates. ( b ) Comparison of observed and predicted BSR biases in G. holbrooki populations. For observed data, the means ±95% confidence intervals are presented. For the predictions, mean and ‘range’ estimates are presented (details in Methods). In both figures, the dotted line represents equal production of sons and daughters. Full size image Males will, depending on their birth season, have mating opportunities with females from either one or two generations ( Figs 2 and 3 ). This selects for male-biased BSRs in spring ( r S ) in ‘anticipation’ of maturation when mating opportunities additionally include females from the preceding generation ( Fig. 4a ). A corresponding ‘anticipatory’ female-biased BSR is expected in the autumn ( r A ). This occurs because autumn-born males, who will breed in spring with only a single cohort of females ( Fig. 3 ), have lower lifetime reproductive output than autumn-born females. Autumn-born males can only fertilize a subset of the total lifetime egg production of females from their generation because some females will outlive the males and breed again the following autumn. These males will still be genetically represented after death as grandparents of the autumn generation. This does not, however, select for the female-biased autumnal sex allocation returning to equality. This is because the grandparental route exists for autumn-born sons and daughters alike. However, only autumn-born daughters can be parents as well as grandparents of some of the zygotes formed 1 year after birth ( Fig. 3 ). Ultimately, the optimal pattern of sex allocation predicted by our model depends only on the degree of female generational overlap ( Fig. 4a ). This is represented by the ratio of available eggs in autumn produced by old, autumn-born females ( E O ) to those from young, spring-born females ( E Y ). These totals encapsulate both the relative abundance of these female classes in autumn as well as their relative fecundities. Our model predicts male-biased BSRs in spring and female-biased BSRs in autumn, with stronger biases as the degree of generational overlap ( E O : E Y ) increases ( Fig. 4a ). When E O is 0 (that is, no generational overlap), a BSR of 0.5 is predicted in both spring and autumn, as predicted by the theory of equal investment [3] , [4] . Estimating generational overlap To parameterize our model, we produced estimates of E O : E Y for each of our study populations by multiplying the numbers of autumn- and spring-born females during the autumn-breeding peak with their predicted fecundities (details in Methods). Incorporation of these fecundity values did not change the ordering of the populations with respect to generational overlap observed in the length distribution of fish. Our estimates (and range) of E O (setting E Y to 1) were: 0.186 (0.109–0.303) for population A, 0.894 (0.658–1.199) for B and 1.665 (1.123–2.470) for C ( Fig. 4a ). BSR of study populations To assess the BSRs produced by female G. holbrooki , we collected 180 pregnant females (30 per population per season) in spring and autumn and sexed the resultant offspring ( N =4,279 offspring, details in Methods; Supplementary Data ). There was a significant mean deviation from an equal BSR in four of the six samples (Wald’s tests for logistic regressions with dispersion parameter set to deviance/df: spring—A: Z =0, P =1, B: Z =2.61, P =0.0091, C: Z =5.274, P <0.0001; autumn—A: Z =−0.98, P =0.33, B: Z =−6.67, P <0.0001, C: Z =−6.47, P <0.0001; Fig. 4b ). The direction of BSR biases differed between seasons, and this difference itself varied across populations (that is, a significant season-by-population interaction), although there was no significant effect of population alone ( Table 1 ). Interestingly, there was also a small but significant effect of maternal body length on BSR (which was consistent across populations and seasons: Table 1 ) with larger females tending to produce more daughters. This result might hint at potential maternal condition-dependent sex allocation [13] , especially as body length is likely to be a more accurate predictor of reproductive output for females than males in G. holbrooki [14] . Table 1 Statistical analysis of G. holbrooki BSRs. Full size table In population A, where there was little female generational overlap ( Fig. 2a ) and weak BSR biases were predicted ( Fig. 4a ), the BSR did not differ from parity in either spring or autumn ( Fig. 4b ). In populations B and C, the BSR was significantly male-biased in spring and female-biased in autumn, and the biases were stronger in population C where the degree of overlap was greatest ( Figs 2b, c and 4b ). Overall, there was a perfect rank-order correlation between the mean observed BSR biases and the mean values predicted by our model when parameterized with field estimates (Spearman’s correlation, ρ 4 =1, P =0.0028). When considering all possible combinations of observed population BSRs and predictions from our model (including mean, upper and lower estimates as per Fig. 4b ), 85.93% produced significant correlations (9 6 combinations, median P =0.017). Given the limited data used to parameterize our model, the fit between predicted and observed patterns of sex allocation is compelling. The sex ratio biases observed were, however, weaker than our model predicted, particularly in spring in populations B and C ( Fig. 3 ). We propose four possible explanations. First, because our estimates of generational overlap ( E O : E Y ) were based on only one breeding season, their long-term (evolutionary relevant) values could be lower if we have overestimated E O or underestimated E Y . For example, because our estimates were based on reproductive output of a sample of pregnant females, variation in the pregnancy rates between seasons might cause a slight bias. If we did overestimate generational overlap, then selection should favour weaker biases than we predicted in all cases. However, because the slope of predicted BSRs is steeper in spring than autumn ( Fig. 4a ), this will lead to a greater reduction in the predicted biases in spring. Future collection of life-history data over longer timescales would allow for more accurate estimates of generational overlap, as well as BSR biases. Second, it is possible that some spring-born females overwintered as adults, but we did not detect them. If so, the asymmetry in generational overlap between female cohorts would be slightly reduced. Third, and similarly, sperm storage by females [15] could effectively create generational overlap for males, if some autumn-born fish are sired using stored sperm from spring-breeding males. Finally, sex allocation might simply be costly to achieve [16] . The observed population differences in female generational overlap are intriguing, given their geographic proximity (<10 km apart). The three artificial reservoirs differ significantly in size but all present similar habitats and predator regimes. Irrespective of the mechanism, however, the high correlation between predicted and observed BSRs suggests that demographic population differences exist. Gene flow between populations is unlikely (human translocation is the only possible mechanism) and Gambusia spp. are known to exhibit rapid evolutionary responses after establishment [17] . Future studies over a wider geographic range would be invaluable in assessing the extent of sex allocation variation in G. holbrooki and the specificity of evolutionary responses. An interesting possibility is that, instead of being a result of micro-evolutionary processes, the patterns of sex allocation observed reflect adaptive plasticity in response to environmental cues of future generational overlap. One could potentially tease these hypotheses apart by attempting to recreate sex allocation biases in a controlled, laboratory environment. Alternative adaptive explanations for the observed seasonal patterns of sex ratio biases are unlikely to apply to our populations. For example, in birds and mammals, seasonal sex ratio patterns can reflect conditional sex allocation when birth date differentially affects the reproductive success of the sexes (for example, if earlier born sons are superior [18] or mature sooner [19] ). For these models to apply to our system, however, all individuals born in spring and autumn would have to compete for the same set of mates at some point in the future. This type of life history is clearly not present here: instead, males only breed once, but with one or two cohorts of females. As with many examples of BSR biases in vertebrates, the proximate mechanisms underlying biases in G. holbrooki remain unknown. They have XX–XY chromosomal sex determination (but might exhibit an overriding autosomal female-determining gene [20] ). General evidence from several taxa suggests, however, that genetic sex determination does not preclude adaptive BSR variation [21] . When considering how many sons versus daughters to produce, it is tempting to focus on parental investment being wasted on offspring that die before reproducing. However, sex differences in mortality do not generally select for greater production of the ‘less wasteful’, better surviving sex. Instead, a decline in the number of surviving adults of one sex simultaneously elevates the reproductive value of each survivor of this sex. This cancelling effect of reproductive value against mortality favours equal investment into sons and daughters. In our study, this perfect cancellation no longer happens as some males (those born in autumn) can only sire a subset of their own cohort’s reproductive output, while others (spring-born males) can sire offspring with females from two age cohorts. This situation creates the opportunity for selection for ‘anticipatory’ adjustment to future mating opportunities. We have provided the first empirical evidence that frequency-dependent selection accounts for changes in sex allocation when future mating prospects vary. Specifically, we show that sex allocation theory can be successfully applied to predict sex ratio adjustment based on temporal shifts in future mating opportunities created by predictable variation in the sex-specific number of cohorts that breed simultaneously. Life-history observations We studied three feral G. holbrooki populations in Canberra, Australia: A—Lake Ginninderra (35.228°S, 149.063°E), B—Lake Burley–Griffin (35.289°S, 149.099°E) and C—Bruce Ponds (35.241°S, 149.091°), from October 2009 to April 2010. We sampled our study populations fortnightly for a total of 12 samples per population. At each sample, we collected fish through both targeted (sweeps directed at visible fish) and random (through submerged and emergent vegetation) dip netting. This was done at two sites per population for 15 min per site to keep catching effort relatively equal. Fish were then separated into males (identified by their gonopodium—modified anal fin), females (identified by a gravid spot near their vent) and juveniles. The males and females were then placed in a shallow container over grid paper and photographed from directly above. These photographs were later used to measure the fishes’ standard lengths, ±0.5 mm, using ImageJ software. The reproductive state (that is, gestating or not) of females was also noted based on the presence/absence of a swollen abdomen. Fish were then returned to the collection site. Analytic model of sex allocation We produced a model of sex allocation tailored to the life history of G. holbrooki populations as outlined above (see Results). First, we consider the optimal BSR in spring ( r S ). The expected mean reproductive output of a son is the number of fertilizable eggs available when he breeds in autumn (contributed by old, E O , and young, E Y , females) shared among all the males that were produced in spring (the product of r S and the number of eggs in spring, E S ): Sons and daughters born in spring both breed once in autumn. This direct reproduction is their only genetic contribution to the population. Natural selection is expected to act on sex allocation so that the expected mean reproductive output of a son and a daughter born in spring is the same: The total number of eggs produced by spring-born females is the product of their expected mean reproductive output and the number of such females: Combining equations (1), (2) and (3) to solve for the BSR in spring yields: Now, we need to calculate the optimal BSR in autumn, r A . These equations are more complicated than those for r S because autumn-born daughters (but not sons) breed twice, thereby overlapping with the spring-born generation. This means that an autumn-born female can make a direct genetic contribution to the next generation of autumn-born fish in a way that an autumn-born male cannot ( Fig. 1 ). Specifically, an autumn-born female can be a mother who breeds the following autumn, as well as a maternal and a paternal grandparent of offspring produced then. Only the latter two types of parentage are possible for an autumn-born male. We can calculate the expected genetic contribution from each of these three possible routes. To obtain the mean expected contribution of an autumn-born male as a grandparent, we note that he can be either a paternal or a maternal grandparent. This male first goes on to sire an expected number of ë S r S sons and (1− r S ) ë S daughters. The expected number of offspring for which he is a paternal grandparent is therefore ë S r S ë A , and the number of offspring for which he is a maternal grandparent is (1− r S ) ë S e Y . We can additionally note the relationship r A ë S =(1− r A ) e S (because of the Fisher condition), which solves to ë S =(1− r A ) e S r A – 1 . Now, using this and equation (2), the expected number of grand-offspring for an autumn-born male simplifies to: Using the same line of reasoning, autumn-born females can be paternal or maternal grandmothers. In spring, these females produce e S r S sons, who then each sire on average ë A offspring. Thus, the expected mean number of grand-offspring obtained as a paternal grandmother is e S r S ë A . Derived similarly, the expected mean number of grand-offspring as a maternal grandmother is e S (1− r S ) e Y . Finally, the expected mean number of ‘grand-offspring equivalents’ that a female zygote formed in the autumn will go on to produce as a mother the following autumn is simply 2 e O . The reproductive output is doubled because a mother is twice as closely related to her offspring than her grand-offspring. Thus, in total, an autumn-born female has the reproductive output e S r S ë A + e S (1− r S ) e Y +2 e O . Again using equation (2), this simplifies to Natural selection is expected to favour a sex ratio that equalizes female and male reproductive output, thus the optimal sex ratio in the autumn is obtained setting This leads to the autumn sex ratio Our final goal is to express r A in terms of the number of available eggs (as these are more tractable parameters than per capita expectations). From the life history ( Fig. 1 ) we know that and that Putting together we now know Now, substituting equation (4) into (3) and solving for e Y , we get Finally, we substitute equations (11) and (12) (which are both expressed in terms of available eggs) into equation (8) to obtain a solution for the BSR in autumn The pattern of sex allocation favoured by natural selection in both spring and autumn therefore depends on the relative number of eggs produced by young (spring-born) and old (autumn-born) females in autumn that are available to be fertilized (that is, the extent of generational overlap for females). Consequently, sex allocation is predicted to be male-biased in spring, and female-biased in autumn ( Fig. 2 ). The strength of the seasonal sex bias increases as the ratio E O : E Y increases (that is, with greater generational overlap), but they asymptote at 1 and 0.25 for spring and autumn, respectively. When E O is 0 (that is, no generational overlap), a BSR of 0.5 is predicted in both spring and autumn, as predicted by Fisher’s theory of equal investment. Estimating generational overlap We parameterized our model using estimates of the number of eggs available to be fertilized in autumn produced by old, autumn-born females ( E O ) and by young, spring-born females ( E Y ). First, we identified young and old females during the autumn reproductive peak (samples 8 and 9) by visual inspection of the length distributions ( Fig. 2 ). Females that could not readily be categorized were excluded. The size ranges used were ≤40 mm (young) and >40 mm (old) for population A, ≤40.5 and >40.5 mm for B, and ≤33 and >33 mm (sample 8) or <33.5 and >35.5 mm (sample 9) for C. Next, we averaged the numbers of these young and old females across samples 8 and 9. Our count estimates were thus 64 (young) and 5 (old) for population A, 65.5 and 17.5 for B, and 40.5 and 34 for C. Next, we estimated the respective fecundities of the two female classes using data from females collected for BSR estimates. We did this by fitting a linear regression of fecundity as explained by female length for each population. We then used these models to predict the mean (±95% confidence interval) fecundities of each generation per population using the mean body length of those females (A: old 31.2 mm and young 46.7 mm, B: 31.8 and 44.8 mm and C: 28.3 and 38.7 mm). This produced mean (and 95% confidence interval) fecundity estimates of 17.3 (young; 13.7–20.9) and 41.2 (old; 29.3–53.2) for population A, 27.1 (23.6–30.6) and 90.7 (75.3–106.1) for B, and 17.0 (13.6–20.4) and 33.7 (27.2–40.2) for C. Next, these estimates of fecundity were multiplied with the respective counts of females to produce estimates for E O and E Y . Finally, a ‘range’ of estimates for E O : E Y were produced by combining the smallest and largest values of E O and E Y , that is, max( E O : E Y )=max( E O ):min( E Y ). BSR of study populations Thirty gestating females were collected from each population during the reproductive peaks in spring and autumn. These females were brought into the laboratory and kept individually until they gave birth. Females that did not give birth within 14 days were replaced. Given a gestation period of 21–28 days, this ensured that sex allocation (assuming it occurs at or around the time of fertilization) occurred while females were in their natural environment. After giving birth, females were euthanized in clove oil solution and measured with dial calipers. Broods were reared in groups of no more than ten in 2 l aquaria at 28 °C on a 14:10 h light:dark photoperiod and fed daily ad libitum . After ∼ 50 days, we sexed and removed individual fry, repeating this every week until all fish were sexed. Sexing was based on anal fin morphology: in males the first few rays of the anal fin fuse during early development of the gonopodium and the anal fin has a concave posterior, while females have anal fins with a convex posterior and unfused rays. Females also begin to develop a gravid spot near their vent. This method of sexing is highly reliable; in a pilot study in which fish were kept in captivity after sexing, 99.1% (209/211) of individuals identified as males were identified correctly and 96.5% (273/283) of individuals identified as females were identified correctly. Mortality during the maturation period was low (16/4297). To be conservative in our analysis, the sex of deceased fry was assumed to be opposite to any BSR bias displayed by the remainder of the brood. Statistical analyses were carried out in R v2.15.0. How to cite this article: Kahn, A.T. et al . Adaptive sex allocation in anticipation of changes in offspring mating opportunities. Nat. Commun. 4:1603 doi: 10.1038/ncomms2634 (2013).